Field-directed sputter sharpening for tailored probe materials and atomic-scale lithography Fabrication of ultrasharp probes is of interest for many applications, including scanning probe microscopy and electron-stimulated patterning of surfaces. These techniques require reproducible ultrasharp metallic tips, yet the efficient and reproducible fabrication of these consumable items has remained an elusive goal. Here we describe a novel biased-probe field-directed sputter sharpening technique applicable to conductive materials, which produces nanometer and sub-nanometer sharp W, Pt-Ir and W-HfB 2 tips able to perform atomic-scale lithography on Si. Compared with traditional probes fabricated by etching or conventional sputter erosion, field-directed sputter sharpened probes have smaller radii and produce lithographic patterns 18–26% sharper with atomic-scale lithographic fidelity. Scanning tunnelling microscopy (STM) facilitates atomic-scale lithography by hydrogen resist patterning; the technique is especially useful for fundamental processes such as patterned oxidation [1] , metallization [2] , [3] , dopant incorporation [4] , templating of organic molecules [5] , [6] and fabrication of quantum cellular automata devices [7] , all at the atomic-scale. Sharpening of probes further extends to field emitters [8] in displays and electron microscopes as well as razor blade manufacturing [9] . Owing to these and other technological applications, numerous methods to effect the sharpening of metallic probes have been developed, several of which involve ion beam processing: sputter erosion sharpening with on-axis inert gas ion beams (conventional sputter erosion (CSE)), self-sputtering with Schiller decapitation [10] and focused ion beam (FIB) sharpening [11] . CSE produces probe radii from 4 nm (ref. 12 ) to ~20 nm (ref. 13 ), and its lower limit has been attributed to surface diffusion processes resulting from thermal and radiation-induced effects [14] , [15] , which in turn depend on ion energy, ion species and substrate material. The Schiller decapitation process creates probes with 4–6 nm radii but offers limited potential for parallel processing due to the need for cutoff detection. FIB sharpening can produce tips with 3–4 nm radii, but remains a serial process requiring skilled oversight. Furthermore, electrochemical etching (ECE) [16] is a common technique for producing probe radii of 10–100 nm. In other cases, researchers have used carbon nanotubes as scanned probes [17] , a challenging serial technique, which provides high resolution at the expense of cost and tailored probe composition. Another collection of techniques focuses on controlling the precise atomic structure of the apex atoms on a probe with limited concern for cone angle and radius of curvature [18] , [19] , [20] . The new technique described here, field-directed sputter sharpening (FDSS), enables both batch fabrication and superior sharpening on the atomic-scale. FDSS eliminates the need for attentive oversight, cutoff detection or fortuitous apex formation and requires only a probe material sufficiently conductive that surface charging is negligible compared with applied probe bias. By fabricating tips composed of HfB 2 , we produce ultra-hard probes capable of stable, high-resolution STM imaging, spectroscopy and patterning. We demonstrate 1 nm radii on platinum-iridium, 2–3 nm radii on tungsten and 4 nm radii on tungsten-hafnium diboride, a substantial improvement over CSE. FDSS methodology In CSE variation of sputter yield with ion angle of incidence is the key factor that enables erosional sharpening [21] , but is insufficient for producing sharp tips on the atomic-scale. This limitation is overcome by FDSS, in which a positive probe bias is applied producing a repulsive potential and localized electric field enhancement at the apex, such that impinging ions are deflected and the effective ion energy upon impact, landing voltage, is the offset between accelerating voltage and probe bias. Ion bombardment of a probe is simulated in two-dimensional space in Fig. 1a , where a uniform Ar ion flux bombards a metallic probe. Because charge accumulation at sharp asperities induces non-uniformity in the electric field, a spatially localized ion deflection potential in the apex region leads to a reduction of ion flux at the probe tip. Our model shows that this flux reduction in the apex region ( Fig. 1b ) follows a square root dependence of average surface ion flux on the ratio of tip bias to ion accelerating voltage ( V r ). In addition, ion angle of incidence is decreased near the probe tip, and surfaces distant from the apex are shielded from sputter erosion. In conjunction with CSE physics, these effects induce enhanced sharpening when compared with grounded-probe CSE sharpening. One prominent reason for this result is reduced ion current density, which leads to a controlled reduction of thermal- and radiation-enhanced surface diffusion in the apex region [22] , [23] , [24] . This FDSS result elucidates the competition between erosional sharpening and diffusion-driven blunting of the tip, which induces an equilibrium curvature that varies with ion flux. Furthermore, the deflection of ions serves to shield the probe taper and shank from further erosion, limiting the influence of FDSS to the crucial apex region without damage to the periphery. FDSS ultimately achieves a dynamic equilibrium in which sputtering continues without modifying the geometry of the tip apex. Although parallel processing of large-tip clusters is limited by the 2 mm ion beam diameter of our apparatus, massively parallel processing could be enabled by a raster scanning ion gun system or by plasma processing. 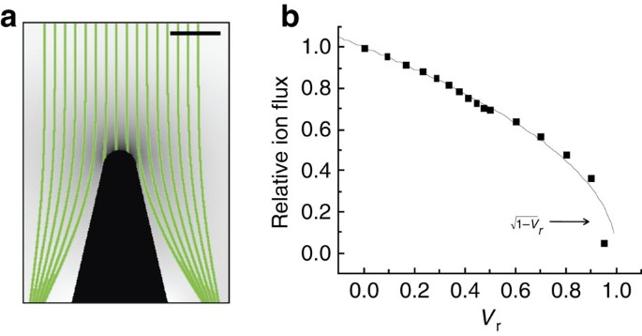Figure 1: Simulation of ion sputtering of a biased probe. (a) Simulated electric field surrounding a two-dimensional probe apex. This model demonstrates the expected field variation with surface curvature and simulated ion flight paths for 1.8 keV singly ionized Ar ions and a probe bias of 800 V (Vr=0.444). Greyscale colouration represents electric field, and green paths represent individual ion paths. Scale bar, 20 nm. (b) Normalized ion current density averaged over a region within 10 nm of the apex centre is shown to exhibit a square root dependence on the ratio of tip voltage to ion accelerating voltage (Vr). An ion flux of 1.0 corresponds to the flux generated at the ion source. Figure 1: Simulation of ion sputtering of a biased probe. ( a ) Simulated electric field surrounding a two-dimensional probe apex. This model demonstrates the expected field variation with surface curvature and simulated ion flight paths for 1.8 keV singly ionized Ar ions and a probe bias of 800 V ( V r =0.444). Greyscale colouration represents electric field, and green paths represent individual ion paths. Scale bar, 20 nm. ( b ) Normalized ion current density averaged over a region within 10 nm of the apex centre is shown to exhibit a square root dependence on the ratio of tip voltage to ion accelerating voltage ( V r ). An ion flux of 1.0 corresponds to the flux generated at the ion source. Full size image Sharpening of platinum-iridium tips A commercial STM tip composed of platinum-iridium alloy (90% Pt, 10% Ir) is sharpened by FDSS. The initial tip has a radius of curvature of 100 nm ( Fig. 2a ). When the probe is bombarded by a 2.0 keV Ne ion beam collinear with the tip axis and a 400 V tip bias is applied ( V r =0.20), sputter erosion causes the probe radius to decrease monotonically (sequence, Fig. 2b ). In its final form, the probe radius of curvature has been reduced to <1 nm ( Fig. 2c ). In this instance, the sharpening process spans 195 min, but in later experiments this time is reduced to 30–60 min by increasing emission current, and therefore, ion flux without modifying the inert gas background pressure. The complete set of transmission electron micrographs (TEM) corresponding to each stage of sharpening is provided in Supplementary Fig. S1 . 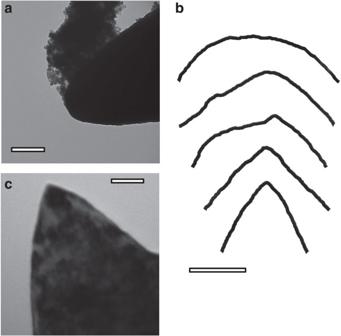Figure 2: Sharpening of a platinum-iridium probe. (a) Transmission electron micrograph of the initial probe, with a 100-nm radius of curvature and significant contaminant adsorption. Scale bar, 100 nm. (b) Apex structure extracted from transmission electron micrographs taken during the sharpening process (2.0 keV ion energy, 400 V probe bias,Vr=0.2). The primary apex is shown as it evolves towards its final form. Between micrographs the probe is sputtered for 75, 60, 30 and 30 min respectively. Required erosion time can be reduced to approximately 30–60 min by increasing ionization rate. Scale bar, 50 nm. (c) The final probe after conclusion of FDSS. The final radius of curvature is below 1 nm. Scale bar, 20 nm. Figure 2: Sharpening of a platinum-iridium probe. ( a ) Transmission electron micrograph of the initial probe, with a 100-nm radius of curvature and significant contaminant adsorption. Scale bar, 100 nm. ( b ) Apex structure extracted from transmission electron micrographs taken during the sharpening process (2.0 keV ion energy, 400 V probe bias, V r =0.2). The primary apex is shown as it evolves towards its final form. Between micrographs the probe is sputtered for 75, 60, 30 and 30 min respectively. Required erosion time can be reduced to approximately 30–60 min by increasing ionization rate. Scale bar, 50 nm. ( c ) The final probe after conclusion of FDSS. The final radius of curvature is below 1 nm. Scale bar, 20 nm. Full size image Sharpening of tungsten tips The reproducibility of FDSS is systematically explored by sharpening of recrystallized [25] W wire in a second, equivalent sharpening system. FDSS is used to sharpen hundreds of recrystallized W probes with 1.5 keV ion energy and 150 V tip bias for 1 h ( V r =0.1), resulting in a typical radius of curvature of 2–3 nm. 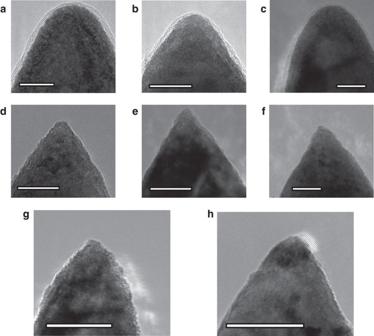Figure 3: Transmission electron micrographs of recrystallized W tips processed by FDSS. (a) TEM image of tip Z1 before sharpening. (b) TEM image of tip Z2 before sharpening. (c) TEM image of tip Z3 before sharpening. (d) TEM image of tip Z1 after sharpening. All tips processed under identical conditions (1.5 keV ion energy,Vr=0.1). (e) TEM image of tip Z2 after sharpening. (f) TEM image of tip Z3 after sharpening. (g) TEM image of tip Z4 after FDSS over a short-time interval (40 min). (h) TEM image of tip Z4 after additional FDSS over a long time-interval (4 h total). All scale bars, 10 nm. Figure 3a–f compares pre- and post-FDSS TEM images of representative W tips that exhibit ultrasharp apices after sharpening under optimized conditions. Tips with this geometry are produced with a yield exceeding 80%. Figure 3: Transmission electron micrographs of recrystallized W tips processed by FDSS. ( a ) TEM image of tip Z1 before sharpening. ( b ) TEM image of tip Z2 before sharpening. ( c ) TEM image of tip Z3 before sharpening. ( d ) TEM image of tip Z1 after sharpening. All tips processed under identical conditions (1.5 keV ion energy, V r =0.1). ( e ) TEM image of tip Z2 after sharpening. ( f ) TEM image of tip Z3 after sharpening. ( g ) TEM image of tip Z4 after FDSS over a short-time interval (40 min). ( h ) TEM image of tip Z4 after additional FDSS over a long time-interval (4 h total). All scale bars, 10 nm. Full size image Figure 3g shows a sharp FDSS W tip after 40 min of sharpening (1.5 keV ion energy, V r =0.1). Following total 4 h of FDSS ( Fig. 3h ), the same tip remains sharp, indicating that sharp W tips do not become blunter with further processing. This allows us to conclude that FDSS is self-limiting and requires less oversight. We also explore the influence of accelerating voltage, tip bias and process time on equilibrium tip geometry. Tip radii produced by FDSS and recrystallized W under different biasing conditions, in contrast to the baseline conditions described above, are shown in Table 1 . We see that the smallest W tip radii are produced with 1.5 keV Ar ion energy and a 150 V tip bias. A set of TEM images from which these data are derived is provided in Supplementary Fig. S2 . In all cases, tips are sharpened and have a single apex; however, sharpness is reduced in comparison to optimized baseline conditions described above. Table 1 Final radius of curvature of recrystallized W tips. Full size table Sharpening of hafnium diboride tips As with CSE, the FDSS technique works with a wide variety of materials, including those for which chemical sharpening techniques are not readily available. One such material is the metallic ceramic hafnium diboride, which can be deposited by conformal chemical vapour deposition (CVD) onto tungsten and other materials [26] , [27] , [28] , [29] . Hafnium diboride possesses material properties that are highly attractive for an STM tip: it is extremely hard (20 GPa in the amorphous state), highly chemically stable and electrically conducting. These characteristics suggest the application of hafnium diboride probes to highly stable microscopy, spectroscopy and electron-stimulated patterning. The probes fabricated in this work exhibit these characteristics, and no adverse effects are observed in topographic and spectroscopic data. Lithographic patterns are similar to those produced by traditional probes of comparable geometry. In this work, amorphous HfB 2 films are grown over ECE and FDSS-sharpened tungsten tips from the carbon-free single-molecular hafnium borohydride precursor, Hf(BH 4 ) 4 , in a low-temperature CVD process. The tip temperature is 290 °C and the growth rate is ~2.5 Å s −1 . The fabrication process is shown schematically in Fig. 4a . Deposition of a nominal 70 nm surface layer of amorphous hafnium diboride affords a probe with a 75-nm radius of curvature ( Fig. 4b ). The absence of a nucleation delay during growth on metallic substrates allows a smooth coating. The composition of the film was probed by energy-dispersive X-ray spectroscopy, shown in Supplementary Fig. S3 . When this tungsten-hafnium diboride probe is exposed to a 1.2-keV Ar ion beam while a 200-V bias is applied to the tip ( V r =0.167), the probe radius is reduced to 4 nm after 60 min ( Fig. 4c ). Because comparable probe radii have been produced from molybdenum wire by CSE [12] , we verify that FDSS significantly improves the radius of our hafnium diboride probe with a control experiment. Further sputtering is performed with the tip unbiased/grounded and the beam energy reduced to 1.0 keV. These conditions were selected to be typical of CSE and to maintain consistent landing voltage when compared with the FDSS experiment. Under these conditions, the radius of the probe increases to 13 nm after 20 min and the apex becomes rougher and asymmetric, as shown in Fig. 4d . We conclude that some of the observed variation in achievable radius of curvature results from choice of material, but that FDSS results in a reduced radius of curvature for each material explored. Another hafnium diboride probe, prepared by the procedure described above, is loaded into an ultrahigh vacuum (UHV) STM for imaging of the Si(100) 2×1:H surface. As imaging probes, sharpened W-HfB 2 tips prove exceptionally stable throughout days of scanning, and provide consistent dimer-resolution imaging as shown in Fig. 5a . The electronic properties of the probe are characterized by constant-spacing scanning tunnelling spectroscopy (STS). The resulting STS data exhibit constant-spacing spectra typical of Si(100) 2×1:H and are remarkably consistent, as revealed by the data set shown in Fig. 5b . 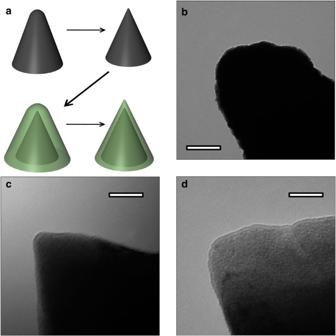Figure 4: Sharpening of a hafnium diboride probe. (a) A schematic representation of the probe growth procedure. An ECE tungsten tip is sharpened by FDSS and a film of amorphous hafnium diboride is grown. The hafnium diboride film is then sharpened by FDSS to bring the tip to its final form. (b) The tip following deposition of a nominal 70 nm amorphous hafnium diboride film. The tip exhibits a radius of curvature of 75 nm and a conformal HfB2coating. Scale bar, 100 nm. (c) After sharpening (1.2 keV ion energy,Vr=0.167, 60 min) the radius of curvature is reduced to 4 nm. Scale bar, 20 nm. (d) As a control, the tip is further sputtered under CSE conditions (1.0 keV ion energy,Vr=0, 20 min). The probe radius increases to 13 nm and the surface exhibits increased roughness and reduced symmetry. Scale bar, 20 nm. Figure 4: Sharpening of a hafnium diboride probe. ( a ) A schematic representation of the probe growth procedure. An ECE tungsten tip is sharpened by FDSS and a film of amorphous hafnium diboride is grown. The hafnium diboride film is then sharpened by FDSS to bring the tip to its final form. ( b ) The tip following deposition of a nominal 70 nm amorphous hafnium diboride film. The tip exhibits a radius of curvature of 75 nm and a conformal HfB 2 coating. Scale bar, 100 nm. ( c ) After sharpening (1.2 keV ion energy, V r =0.167, 60 min) the radius of curvature is reduced to 4 nm. Scale bar, 20 nm. ( d ) As a control, the tip is further sputtered under CSE conditions (1.0 keV ion energy, V r =0, 20 min). The probe radius increases to 13 nm and the surface exhibits increased roughness and reduced symmetry. Scale bar, 20 nm. 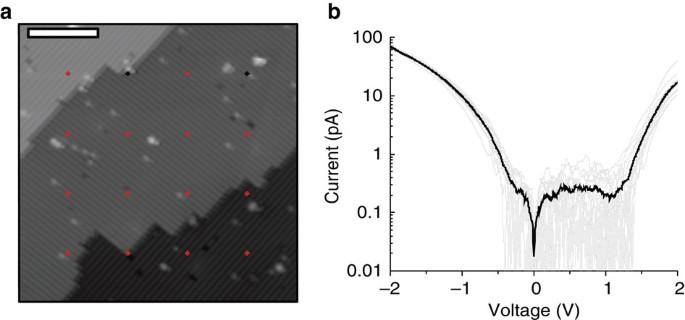Figure 5: STM and constant spacing STS of the Si(100) 2×1:H surface using W-HfB2STM tips. (a) STM image demonstrating high stability and consistent dimer row resolution, with the locations of STS data collection denoted in red. Black crosshairs represent data points, which were excluded due to the presence of a dangling bond directly beneath the probe. Topographic data were collected with a sample bias of −2 V and current set point of 50 pA. Scale bar, 10 nm. (b) STS data on a semi-log plot. The average of the 14 spectra points is shown in black, with the individual spectra shown in grey. Full size image Figure 5: STM and constant spacing STS of the Si(100) 2×1:H surface using W-HfB 2 STM tips. ( a ) STM image demonstrating high stability and consistent dimer row resolution, with the locations of STS data collection denoted in red. Black crosshairs represent data points, which were excluded due to the presence of a dangling bond directly beneath the probe. Topographic data were collected with a sample bias of −2 V and current set point of 50 pA. Scale bar, 10 nm. ( b ) STS data on a semi-log plot. The average of the 14 spectra points is shown in black, with the individual spectra shown in grey. Full size image Electron-stimulated desorption lithography STM can be used to effect the electron-stimulated desorption (ESD) of hydrogen from silicon [1] , [30] , [31] , providing a lithographic mask for subsequent deposition. Hydrogen desorption patterning can be achieved at the atomic-scale [32] , [33] with a low patterning rate (vibrational heating). However, increased throughput can be achieved for higher electron energy, and therefore higher desorption yield (direct electronic excitation). Because a single inelastic electron scattering event is sufficient to modify the Si:H surface under direct electronic excitation, the spatial distribution of the tunnelling current between tip and sample becomes a significant factor in pattern fidelity [34] , [35] . As probes with a smaller radius of curvature enable higher resolution lithography [34] , we therefore expect FDSS-processed probes to enable superior tip-based nanolithography. We demonstrate this result by ESD of hydrogen from Si(100) using tungsten tips generated by three methods: FDSS, ECE and CSE. The lines patterned by FDSS probes have consistently higher resolution than those patterned by ECE and CSE probes. In this experiment, a single polycrystalline tungsten probe is sequentially sharpened by all three methods, and following each method the probe is used for ESD of hydrogen from a Si(100) 2×1:H surface. When the tip is sharpened by ECE, the initial apex ( Fig. 6a ) has a 5±1 nm radius of curvature (11.5±0.5 nm oxide radius). The probe is then degassed above 400 °C for 8 h in UHV and used repeatedly to write a series of lithographic lines ( Fig. 6b ). The tip is then removed from the STM and sharpened by FDSS. From a TEM image ( Fig. 6c ) the tip radius is 2±1 nm (5.5±0.5 nm oxide radius). After the TEM study, the tip is reinserted into our vacuum system and resharpened by FDSS under identical conditions to remove native oxide. After the probe is degassed above 400 °C for 8 h, it is again used to write a series of lithographic lines ( Fig. 6d ). Imaging and patterning resolution improve markedly. 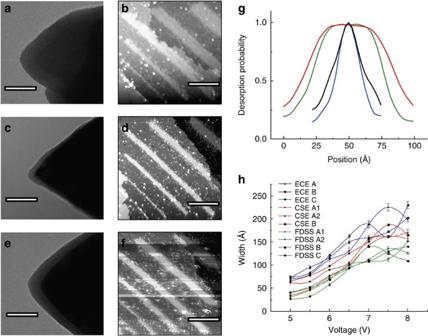Figure 6: Effects of probe sharpening on patterning capabilities. Each hydrogen-resist pattern includes a sequence of lines corresponding to sample biases from lower left to upper right of 4, 4.5, 5, 5.5, 6 and 6.5 V with constant tunnelling current of 2 nA and line dose of 2×10−3C cm−1. STM images are collected with a sample bias of −2 V and a current set point of 50 pA. All scale bars, 30 nm. (a) Transmission electron micrograph of an exceptionally sharp tungsten probe produced by ECE. (b) A representative pattern on the Si(100) 2×1:H surface written by electron-stimulated desorption of hydrogen using the ECE probe ofa. (c) Transmission electron micrograph of the probe following an FDSS sharpening procedure (1.4 keV ion energy,Vr=0.286, 38 min). (d) A representative pattern created with this FDSS-generated probe. (e) Transmission electron micrograph of the same probe following control experiment sputtering (1.0 keV ion energy,Vr=0, 60 min). (f) A representative pattern created with the control probe. (g) Spatial distribution of desorption probability for FDSS and CSE probe patterns at 5.5 and 4.5 V sample bias. In order of decreasing width, CSE 5.5 V pattern is shown in red, FDSS 5.5 V pattern in green, CSE 4.5 V pattern in black and FDSS 4.5 V pattern in blue. (h) Further patterning results from multiple probes sharpened by ECE, FDSS and CSE. Figure 6: Effects of probe sharpening on patterning capabilities. Each hydrogen-resist pattern includes a sequence of lines corresponding to sample biases from lower left to upper right of 4, 4.5, 5, 5.5, 6 and 6.5 V with constant tunnelling current of 2 nA and line dose of 2×10 −3 C cm −1 . STM images are collected with a sample bias of −2 V and a current set point of 50 pA. All scale bars, 30 nm. ( a ) Transmission electron micrograph of an exceptionally sharp tungsten probe produced by ECE. ( b ) A representative pattern on the Si(100) 2×1:H surface written by electron-stimulated desorption of hydrogen using the ECE probe of a . ( c ) Transmission electron micrograph of the probe following an FDSS sharpening procedure (1.4 keV ion energy, V r =0.286, 38 min). ( d ) A representative pattern created with this FDSS-generated probe. ( e ) Transmission electron micrograph of the same probe following control experiment sputtering (1.0 keV ion energy, V r =0, 60 min). ( f ) A representative pattern created with the control probe. ( g ) Spatial distribution of desorption probability for FDSS and CSE probe patterns at 5.5 and 4.5 V sample bias. In order of decreasing width, CSE 5.5 V pattern is shown in red, FDSS 5.5 V pattern in green, CSE 4.5 V pattern in black and FDSS 4.5 V pattern in blue. ( h ) Further patterning results from multiple probes sharpened by ECE, FDSS and CSE. Full size image As an experimental control, the tip is then sputtered under CSE conditions with a 1.0 keV ion beam and a grounded probe. Inspection via TEM ( Fig. 6e ) shows that the radius of curvature has increased to 8±1 nm (12.0±0.5 nm oxide radius). The tip is further sputtered under identical conditions to eliminate native oxide and is again degassed above 400 °C for 8 h before additional patterns are written. Imaging resolution is reduced; tip instability is enhanced, as indicated by multiple tip changes within the image; and pattern width increases ( Fig. 6f ). The reproducibility of pattern writing is also markedly better for FDSS-sharpened probes than ECE probes ( Supplementary Fig. S4a ). This improvement largely results from the removal of chemisorbed and physisorbed species during sputtering, but also addresses concerns about tip instability resulting from ion-induced radiation damage. Even in the absence of a high-temperature anneal, typical FDSS probes provide immediate stable dimer resolution imaging. It is noteworthy that our ECE probe appears exceptionally sharp as judged by TEM (above the 95th percentile of ECE tungsten tips from our facility). This makes our observation of improvement following FDSS even more significant. Hydrogen resist patterns produced by FDSS probes have reduced line widths compared with those written by both ECE and CSE probes. The FDSS probe generates line widths of 2.2 nm for 4.5 V patterns and 5.8 nm for 5.5 V patterns. By comparison, the ECE probe generates 2.8 and 7.9 nm patterns, whereas the control probe generates 2.7 and 7.3 nm patterns. Thus, the FDSS patterns exhibit a 21% (4.5 V) and 26% (5.5 V) reduction in line width over the ECE probe and an 18% (4.5 V) and 20% (5.5 V) reduction in line width over the control probe. This reduction in patterning width is found to be statistically significant by a two-tailed Welch's t -test ( α =0.10). A comparison between FDSS and CSE patterns for both 4.5 V and 5.5 V patterns is presented in Fig. 6g , and further data are provided in Supplementary Fig. S4b,c . Comparing ECE and CSE probes, we cannot reject the null hypothesis for 4.5 V ( P =0.50) or 5.5 V ( P =0.65) sample bias, allowing for the possibility that CSE offers no improvement over a sharp ECE probe. In a subsequent experiment, we verify the reproducibility of these results across multiple STM tips, and across multiple tip sputtering cycles. A set of three ECE probes, with a range of apex radii, are selected by TEM (micrographs are shown in Supplementary Fig. S5 ) as clean and potentially stable STM tips. The tips are sharpened and patterns written using the process described above, with sample biases from 4 to 8 V. Each tip is sharpened by FDSS (1.4 keV beam voltage, V r =0.286) and after patterning, sputtered under CSE conditions (1.0 keV beam voltage, V r =0). Tip C received damage unrelated to sputtering and scanning before the control experiment, but ECE and FDSS data are shown for completeness. Tip A was FDSS sharpened a second time after control patterning, and a second control experiment completed. The resulting pattern widths are shown in Fig. 6h , where we see a clear and reproducible reduction in pattern width as we move from ECE tips to CSE tips and finally to FDSS tips for which optimal resolution is achieved. It is noteworthy not only that each tip exhibits improved patterning after FDSS, but also that the images collected after FDSS achieve atomic resolution imaging from the very first scan ( Supplementary Fig. S6 ). Furthermore, the cycling of tip A through multiple FDSS and control cycles further demonstrates the reproducibility of FDSS not only from one tip to the next, but also for a single tip over multiple sputtering cycles. Using tungsten tips sharpened by FDSS, we are able to effect ultrahigh fidelity patterning of Si(100) 2×1:H surfaces by ESD. An ECE tungsten tip is first sputtered by 1.2 keV argon ions while a 200 V probe bias is applied, and the resulting probe is used to generate several lithographic patterns ( Fig. 7 ), including a dimer row periodic structure and a two-dimensional nanobox. The periodic structure is generated by two successive 4 V patterning cycles and represents the smallest lithographic pitch demonstrated in this work: the lines are separated by the width of a single silicon dimer row. To generate the nanobox, five successive patterning cycles are completed, resulting in an extremely high fidelity 20×13 atom box. Most of the peripheral dangling bonds were present before patterning, but occasional spurious depassivation events can occur outside the bounds of a mask, and may result from electron backscattering [36] . These spurious events occur less frequently with tungsten FDSS probes than with hafnium diboride probes, but further characterization is necessary to quantify and explain the relation between probe geometry, probe composition and spurious depassivation. As an example of this relationship, the patterns in Fig. 7 can be compared with that shown in Supplementary Fig. S7 , in which a W-HfB 2 probe (6 nm radius) is used for patterning, and more spurious dangling bonds are generated. 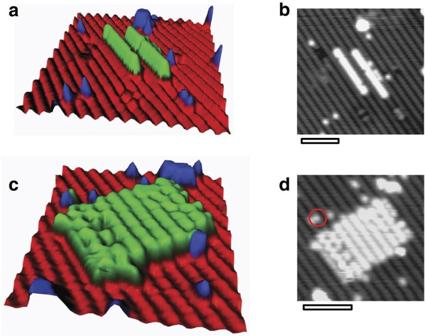Figure 7: Demonstration of atomic-fidelity lithography by ESD. Shown is the ESD of hydrogen from the Si(100) 2×1:H surface with a 4-V sample bias, a 2-nA current set point, 2×10−3C cm−1line dose and FDSS-generated tungsten probe. STM images are collected with a sample bias of −2 V and a current set point of 50 pA. All scale bars, 4 nm. (a) Dimer-row line width lithography is demonstrated. The image is a false-colour three-dimensional rendering where red represents passivated silicon, blue represents background surface features unrelated to patterning and green represents dangling bonds generated by the ESD process. (b) The same pattern is shown in its original form as a two-dimensional STM topograph. (c) A nanolithographic box 20×13 atoms in dimension is shown as a false-colour three-dimensional rendering similar to that ina. The feature has been generated by five successive depassivation patterns under identical patterning conditions. (d) Topographic STM data in two-dimensions is also shown for the nanobox pattern. Figure 7: Demonstration of atomic-fidelity lithography by ESD. Shown is the ESD of hydrogen from the Si(100) 2×1:H surface with a 4-V sample bias, a 2-nA current set point, 2×10 −3 C cm −1 line dose and FDSS-generated tungsten probe. STM images are collected with a sample bias of −2 V and a current set point of 50 pA. All scale bars, 4 nm. ( a ) Dimer-row line width lithography is demonstrated. The image is a false-colour three-dimensional rendering where red represents passivated silicon, blue represents background surface features unrelated to patterning and green represents dangling bonds generated by the ESD process. ( b ) The same pattern is shown in its original form as a two-dimensional STM topograph. ( c ) A nanolithographic box 20×13 atoms in dimension is shown as a false-colour three-dimensional rendering similar to that in a . The feature has been generated by five successive depassivation patterns under identical patterning conditions. ( d ) Topographic STM data in two-dimensions is also shown for the nanobox pattern. Full size image The high-fidelity patterning capabilities of FDSS-prepared probes can persist over many hours of scanning and patterning, but as with any STM tip, ultimately probe quality will degrade. The FDSS process is well suited for regeneration of damaged probes, and in cases where damage is on the sub-micron scale high-resolution patterning capabilities can be fully recovered ( Supplementary Fig. S8 ). As the size of the probe increases, so does the time required for sharpening, suggesting that resharpening of extremely blunt probes is impractical, although not impossible. In this paper, we have demonstrated the efficacy and reproducibility of FDSS and explored its use in the fabrication of tailored probe materials. The generality of this technique is of particular importance. Through the sharpening of tailored thin films, a wide range of mechanical, electrical, optical and catalytic material properties can be explored and exploited. Second, the potential for massively parallel FDSS makes it unique among sharpening techniques of this kind. Techniques comparable in sharpening efficacy (for example, FIB and carbon nanotubes) do not presently offer the same degree of parallelizability. Finally, FDSS offers a significant reduction in radius of curvature when compared with earlier sputter sharpening techniques. The fabrication of a 1-nm radius probe, beyond the last atoms, is a remarkable result, and the high yield and reproducibility of FDSS offers promise for widespread implementation. In conclusion, FDSS offers a significant step towards the production of metallic probes of ultimate sharpness. In particular, we have shown how ultra-hard HfB 2 offers W tips increased fidelity and stability for high-resolution STM and STS. Given the simplicity of the sharpening recipe and dependence only upon equipment already common within many laboratories, FDSS can be immediately applied to a large and continually expanding collection of experimental and industrial processes. The reliability of the technique, and potential for high throughput, offers exciting opportunities for highly parallelized tip-based nanofabrication moving towards the limit of atomically precise manufacturing. Tip etching and sputter sharpening Tungsten probes are prepared by drop-off (lamellae) ECE in NaOH. After rinsing in deionized water they are sharpened by FDSS before optional hafnium diboride deposition. Platinum-iridium probes are purchased from Materials Analytical Services. During transportation, atmospheric exposure is minimized and electrostatic discharge-safe practices are employed. Sputter sharpening is performed in a turbo-pumped high-vacuum antechamber with a background pressure below 5×10 −8 Torr. During sputter erosion, neon or argon is flowed through a variable leak valve to achieve a pressure of 5.5×10 −5 Torr, the probe potential is controlled by a high-voltage (0–1 kV) DC power supply and the ion beam is generated by a Physical Electronics PHI 04-161 integrated ion source with a nominal beam diameter of 2 mm. The sample is held at a distance of 5–10 cm from the focusing assembly. The sample temperature is not controlled. For tips that oxidize before TEM imaging, we approximate the achievable probe radius from the radius of a native oxide layer and of the sub-surface tungsten core. Probes are loaded into the STM after sputter sharpening without atmospheric exposure. HfB 2 chemical vapour deposition Deposition of hafnium diboride film is performed in a turbo-pumped high-vacuum chamber with a background pressure below 5×10 −8 Torr. During deposition, the probe is heated and exposed to Hf(BH 4 ) 4 precursor. Film thickness is measured on an adjacent silicon wafer by ellipsometry during growth and verified by transmission electron microscopy of the STM tip. STM and surface preparation Passivation and STM are performed in an UHV chamber with a background pressure below 1×10 −10 Torr. Scanning and patterning are performed at room temperature in a home-built UHV-STM system [37] . The Si(100) 2×1:H surface is prepared by overnight degas at 600 °C followed by three 1,250 °C flashes (30 s, 10 s, 5 s) and passivated by atomic hydrogen generated at a 1,300 °C tungsten filament in a hydrogen background (2×10 −6 Torr). During passivation, the sample is held at 377 °C for 10 min (1,200 L dose) at a distance of 5–10 cm from the tungsten filament. During electron-stimulated hydrogen desorption, the sample bias is held constant, whereas computer control adjusts the tip height to maintain the designated tunnelling current (2 nA). Tip velocity is set appropriately to maintain a 2×10 −3 C cm −1 line dose (100 Å s −1 ). To extract desorption probability across a line profile, the topographic height is averaged along the length of a line (or that portion predominantly unaffected by tip instability during imaging) and scaled linearly to the zero to one range. This technique averages out random deviations due to surface defects and background dangling bonds, and provides an accurate approximation of desorption probability in cases where the desorption probability peak very closely approximates unity, as is the case in this experiment. Line width is defined as the full-width at half-maximum of desorption probability. Ion flux simulations Ion paths are simulated by an iterative electric potential computation with a 2.5-Å square mesh. The potential is computed with an iterative Poisson solver by the Jacobi method. We apply a zero-field condition at the left and right boundary, and fix the electric potential to ground and tip bias at the upper and lower boundaries, respectively. The ion path is computed deterministically within each mesh point ( F = ma ), and computed recursively until an ion impacts or escapes the system. The average ion current density is computed by assuming a uniform ion flux at the source and determining the spatial limits of ion initial position that permit impact within the area of interest on our probe. How to cite this article: Schmucker, S.W. et al . Field-directed sputter sharpening for tailored probe materials and atomic-scale lithography. Nat. Commun. 3:935 doi: 10.1038/ncomms1907 (2012).